Catalytic activation of pre-substrates via dynamic fragment assembly on protein templates Sensitive detection of small molecule fragments binding to defined sites of biomacromolecules is still a considerable challenge. Here we demonstrate that protein-binding fragments are able to induce enzymatic reactions on the protein surface via dynamic fragment ligation. Fragments binding to the S1 pocket of serine proteases containing a nitrogen, oxygen or sulphur nucleophile are found to activate electrophilic pre-substrates through a reversible, covalent ligation reaction. The dynamic ligation reaction positions the pre-substrate molecule at the active site of the protein thereby inducing its enzymatic cleavage. Catalytic activation of pre-substrates is confirmed by fluorescence spectroscopy and by high-performance liquid chromatography. The approach is investigated with 3 pre-substrates and 14 protein-binding fragments and the specific activation and the templating effect exerted by the enzyme is quantified for each protease–fragment–pre-substrate combination. The described approach enables the site-specific identification of protein-binding fragments, the functional characterization of enzymatic sites and the quantitative analysis of protein template-assisted ligation reactions. Fragment-based development of protein ligands has been recognized over the last years as a powerful strategy to identify molecules with an optimized fit to protein-binding pockets, providing ligands with reduced molecular weight and with higher ligand efficiency, thereby possibly improving the bioavailability, cell permeability and metabolic stability of drug molecules [1] , [2] , [3] , [4] , [5] , [6] , [7] , [8] . Scrutinizing the chemical space of small molecule fragments—instead of screening large libraries of drug-like molecules—requires considerably smaller chemical libraries for covering the chemical space and thus enables to identify and optimize hit ligands with less effort for testing and chemical synthesis. There are, however, specific challenges implicated in the fragment-based drug discovery process. Many primary fragment hits possess low, often millimolar affinities to the protein target resulting from the small contact area and the low number of binding interactions of fragments compared with larger molecules. As a consequence, high concentrations of fragments have to be used in the bioassays, which can interfere with the reliable read-out of classical biochemical test systems. To circumvent this problem, biophysical methods have been employed for the detection of protein-binding fragments, using, for example, nuclear magnetic resonance (NMR) spectroscopy [9] , [10] or X-ray diffraction of protein crystals [11] , [12] , [13] , [14] . Next, primary fragment hits with low affinity have to be extended to fragment combinations to attain sufficient activity—a process requiring the systematic modification of hits by applying tools and methods of medicinal chemistry. Realistically, this optimization process can be more time-consuming and uncertain in its outcome than the initial discovery of fragment hits. Fragment combinations have been synthesized and tested not only for direct inhibitor screening, but also for the screening of substrate libraries. Active substrates can then serve as a starting point for the development of enzyme inhibitors following a seminal concept in medicinal chemistry [15] , [16] . Dynamic ligation screening (DLS) has been introduced as an approach for the sensitive, site-selective detection of protein-binding fragments [17] . In this method, a chemically reactive protein ligand serves as a directing probe for the screening of fragment libraries at a spatially defined protein site [18] . Reversible formation of a covalent bond between the directing probe and a nucleophilic fragment enables the sensitized detection of low-affinity fragments with millimolar activity while testing at lower concentrations of 10–100 μM. This sensitizing effect results from the templated assembly of protein ligands on the protein surface. As a consequence, standard biochemical assays can be applied for the detection of low-affinity fragments, for example, the enzymatic conversion of a fluorogenic substrate or fluorescence polarization for a binding assay [19] . DLS provides fewer hits than biophysical assays, as only fragments with a fitting spatial orientation in the ligation product are detected as actives. Active fragment combinations were identified and optimized iteratively, with respect to affinity or, if second-site-specific fragments are scrutinized with sets of proteins, with respect to specificity [20] . Other than in biophysical assays, nanomolar protein concentrations are sufficient and large collections of nucleophilic fragments can be tested in small volumes of liquids on microtitre plates. Conceptually, DLS constitutes a specific application of dynamic covalent chemistry, which has been defined as that branch of organic chemistry studying compounds formed reversibly in thermodynamic equilibrium [6] , [21] . Therefore in principal all dynamic ligation reactions should be applicable to fragment ligation assays, yielding, for example, imines [22] , [23] , [24] , hydrazones [25] , [26] , hemiacetals [27] , [28] , hemithioacetals [29] , acetals [30] , [31] , thioesters [32] or Michael addition products [33] . In this paper we wish to explore a novel approach for the identification of protein-binding fragment assemblies formed by dynamic covalent chemistry introduced here as the ‘pre-substrate concept’. Central idea of this approach is to employ completely inactive reporter probes denominated as ‘pre-substrates’ for the detection of protein-binding fragments and/or to use such probes for the detection or discovery of hitherto unknown reactive sites on protein surfaces. Pre-substrates are supposed to contain a reactive site, for example, an electrophile like aldehyde or Michael acceptor moiety for covalent ligation with various nucleophiles and an N- acylated reporter dye such as the fluorophore 7-amino-4-methylcoumarin (AMC) for detection. As N -deacylation of the acylated 7-amino group in AMC shifts the fluorescence emission of the coumarin dye to longer wavelengths, the cleavage of this amide bond by a hydrolytic enzyme is detectable as a time-dependent increase in fluorescence. In this contribution we demonstrate that electrophilic pre-substrates are valuable tools for the detection of biologically active fragments in a fluorescence-based enzyme assay and that the assay system enables the quantification of the templating effect exerted by the target protein for each fragment–pre-substrate combination. The concept of pre-substrate activation To establish the assay system, serine proteases were selected as model targets ( Fig. 1 ). Nucleophilic fragments, which bind to the S1 substrate-binding pocket of a serine protease were expected to assemble with a pre-substrate in a protein-templated reaction under formation of a covalent bond between the fragment nucleophile with the electrophile of the pre-substrate. In case of an optimal fit to the protein, this fragment assembly should position the amide bond of the pre-substrate at the active site of the protein and thus induce cleavage of the pre-substrate by the enzyme, which would result in the release of the coumarin fluorophor and generate a time-dependent increase in fluorescence. The experimental set-up should enable the parallel testing of several fragments, for example, in microtitre plates. Determination of the rate of the enzymatic reaction and its concentration-dependent saturation will then allow us to determine the stability of the enzyme–substrate complex (apparent K M ) consisting of a protease, the S1-binding nucleophile fragment and the pre-substrate. The recorded K M values reflect the thermodynamic stabilization of the fragment–pre-substrate–enzyme complex (through K M ≤K D and G ≤ RT ln K M ) and thereby quantify the templating effect exerted by the enzyme, resulting in the shift of the ligation equilibrium. Thereby, the pre-substrate concept will enable the quantitative analysis of dynamic ligation reactions of nucleophiles and electrophiles on protein templates. 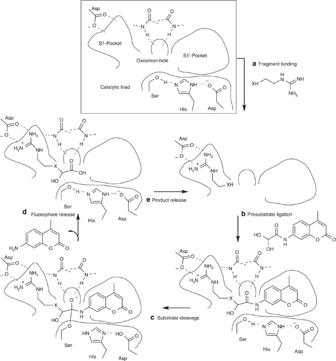Figure 1: The concept of pre-substrate activation by protein-binding fragments. Fragments bind to the S1 pocket of trypsin-like proteases with reported affinity (a). Only in case where the nucleophile is positioned correctly, ligation of a pre-substrate occurs (b), resulting in cleavage (c) of the formed substrate and release of the cleavage products (d,e). Figure 1: The concept of pre-substrate activation by protein-binding fragments. Fragments bind to the S1 pocket of trypsin-like proteases with reported affinity ( a ). Only in case where the nucleophile is positioned correctly, ligation of a pre-substrate occurs ( b ), resulting in cleavage ( c ) of the formed substrate and release of the cleavage products ( d , e ). Full size image N -Glyoxalyl-AMC 1 was designed and synthesized as the first potential pre-substrate, ( Fig. 1 , Supplementary Fig. 1 ). In aqueous solution, 1 is hydrated as indicated by the corresponding acetal proton at 5.99 pm in the 1 H-NMR in acetone/D 2 O and by the absence of the aldehyde proton, which can be observed at 10.08 ppm in dimethyl sulfoxide (DMSO) solution. Hydration of 1 is favoured thermodynamically in aqueous solution due to the electrophilicity of 1 and due to the high concentration of the water nucleophile (55 M). As a result, at physiological pH of 7.4 the equilibrium of ligation reactions of 1 with most O- , N- or S- nucleophiles providing hemiacetals, imines or thiohemiacetals as ligation products is on the side of the hydrate—with few exceptions like aromatic amines. We hypothesized, however, that despite the favoured hydration of 1 , a templating effect exerted by a fitting protein surface might still enable the formation of fragment ligation products of 1 and a nucleophile. If these ligation products can be formed, they might position the amide bond of 1 in the active site of the enzyme and thereby induce the cleavage of the pre-substrate. Thus, observing amide bond cleavage of 1 will prove both the covalent ligation of both fragments and the templating effect of the protein surface. As target proteins, two serine proteases were selected, factor Xa (FXa) and trypsin, two enzymes with well-described preferences for substrate recognition in the S1 pocket, which is adjacent to the protein’s active site and thus might be accessible by fragments ligated to the aldehyde position of 1 . The first target, FXa, is a key-player in the blood coagulation cascade and an established drug target for inhibition of haemostasis. It prefers to cleave substrates with arginine (Arg) next to the cleavage site [34] . The second target, trypsin, not only hydrolyzes peptides with arginine at P1, but also those endowed with lysine (Lys) at the cleavage site and plays its major role in digestion in the duodenum [35] . While trypsin has a broad substrate tolerance, FXa has rather specific substrate requirements. Proof-of-concept It was attempted to prove the validity of the pre-substrate concept with respect to the potential pre-substrate 1 ( Fig. 2 ). The small peptide substrate Boc-Leu-Gly-Arg-AMC or the shortened amino acid substrate Z-Arg-AMC were incubated with one of the proteases (3.5 nM) in a 50 mM 3-( N -morpholino)propanesulfonic acid buffer (MOPS buffer) at pH 8 and room temperature. For both enzymes a distinct increase in fluorescence was recorded indicating the efficient turnover of both substrates. Next, the potential pre-substrate 1 was incubated with one of the proteases under the same conditions. Even at concentration up to 12.6 mM absolutely no conversion of 1 was recorded and thus 1 was proven not to be a substrate of either trypsin or FXa. 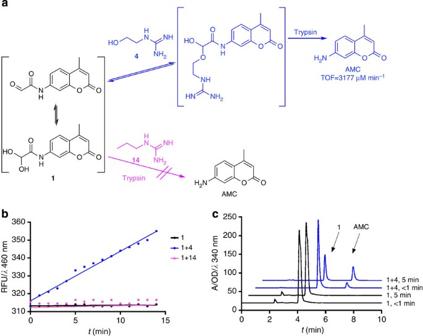Figure 2: Proof-of-concept. Pre-substrate1was completely inactive towards cleavage with trypsin (a, black). Addition of fragment4, a ligand that binds to the S1 pocket of trypsin, resulted in the activation of the pre-substrate, cleavage of the amide bond and the release of the reporter dye 7-amino-methyl coumarin (AMC;a, blue). No fluorescence was emitted in the presence of negative control fragment14(a, magenta). Formation of AMC was followed by fluorescence spectroscopy (b) and HPLC (c) and can be rationalized by formation of a hemiacetal ligation product and its recognition by the protein. The experiments were replicated twice by two different operators with duplicate repeated measures within each replication. Each data point represents the average of double determination. Figure 2: Proof-of-concept. Pre-substrate 1 was completely inactive towards cleavage with trypsin ( a , black). Addition of fragment 4 , a ligand that binds to the S1 pocket of trypsin, resulted in the activation of the pre-substrate, cleavage of the amide bond and the release of the reporter dye 7-amino-methyl coumarin (AMC; a , blue). No fluorescence was emitted in the presence of negative control fragment 14 ( a , magenta). Formation of AMC was followed by fluorescence spectroscopy ( b ) and HPLC ( c ) and can be rationalized by formation of a hemiacetal ligation product and its recognition by the protein. The experiments were replicated twice by two different operators with duplicate repeated measures within each replication. Each data point represents the average of double determination. Full size image Next, 1 (3 mM) was incubated in the very same assay with trypsin (3.5 nM) and a strong excess of N -(2-hydroxyethyl)guanidine 4 (7.7 mM) as a potentially activating nucleophilic fragment. 4 was selected for this purpose as it was expected to bind to the S1 site of the protein and could be able to form an isosteric ligation product with 1 , which might position the AMC-amide bond at the active site of the protease. Indeed, the mixture of 1 and 4 with each of the proteases produced a time-dependent, linear increase in fluorescence at 460 nm ( Fig. 2b ). The observed effect depended critically on the presence of the protease: pre-substrate 1 and fragment 4 in buffer without addition of the protease did not affect cleavage of 1 and an increase in fluorescence. For another negative control, the non-nucleophilic control fragment propyl guanidine 14 was incubated with 1 and the protease at high concentrations. No cleavage of the pre-substrate was observed under these conditions, either. This experiment excludes the theoretical possibility that the guanidine fragment can induce cleavage of the pre-substrate by binding to S1 without ligating to the pre-substrate. For a secondary and independent confirmation of pre-substrate activation, the reaction mixture consisting of pre-substrate 1 (0.3 mM), trypsin and bis-nucleophilic fragment 4 (2-aminoethanol) was analyzed by high-performance liquid chromatography (HPLC) at different time points. The fluorescence increase at 430 nm was found to correlate with cleavage of the amide bond in 1 and the release of non-acylated AMC ( Fig. 2c , Supplementary Fig. 8 ). Additionally, possible side reactions of pre-substrate 1 with side chains of trypsin were excluded using MALDI-ToF/ToF mass spectrometry ( Supplementary Figs 9–11 ). In summary, these experiments confirmed that pre-substrate 1 , which was completely inactive towards the protease alone, was activated by covalent dynamic ligation with nucleophile 4 . Potential pre-substrates and fragments The scope of the pre-substrate concept was to be investigated with respect to the selection of nucleophiles, which undergo the activating ligation reaction, and with respect to the pre-substrates to be used. In addition to the first pre-substrate, N -glyoxalyl-AMC 1 (2-oxo- N -(4-methyl-2-oxo-2H-chromen-7-yl)-acetamide), N -malonalyl-AMC 2 (3-oxo-( N -(4-methyl-2-oxo-2H-chromen-7-yl)-propanoylamide) and N -acryloyl-AMC 3 ( N -(4-methyl-2-oxo-2H-chromen-7-yl)-acrylamide) were designed as potential alternatives ( Fig. 3 , Part a). In pre-substrate 2 a methylene bridge was inserted between the acyl-AMC and the aldehyde functionality, resulting in fragment ligation products elongated by one carbon. In addition, the CH acidity at C2 of the malonyl aldehyde should facilitate the enolization and thereby might favour the formation of ligation products compared with 1 . Acrylamide 3 was chosen to test the possibility of Michael additions with nucleophiles potentially yielding bioactive substrate structures. Both compounds 2 and 3 were completely stable towards both proteases under assay conditions without nucleophilic fragments, establishing them as pre-substrates. A small collection of 14 fragments ( 4–17 ) was composed containing various N- , O- and S- nucleophiles (amines, alcohols and mercaptanes) and non-nucleophilic control fragments as potential mimetics of the arginine or Lys side chains ( Fig. 3 , Part b). The already mentioned N -(2-hydroxyethyl)guanidine 4 was complemented by its amino- and mercapto-derivatives ( 5 , 6 ), the diamines 7 and 8 as potential mimetics of the Lys side chain were complemented by ethanolamine 9 and 2-mercaptoethanamine 10 . 4-(aminomethyl)benzamidine 11 , 4-aminobenzamidine 12 and aminoguanidine 13 represent further classical mimetics of the arginine side chain. N -propylguanidine 14 , S -ethylisothiourea 15 and propylamine 16 were selected as negative controls, while 5-chloro-2-thiophenemethanol 17 was included as the fragment binding to the S1 pocket of FXa in the drug rivaroxaban ( Fig. 3 , Part b). 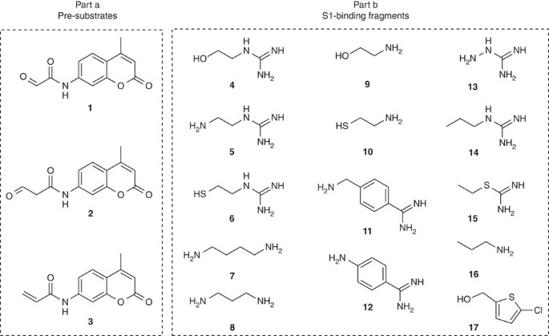Figure 3: Structure of potential pre-substrates 1–3 and S1-binding fragments 4–17. The details of the synthesis of compounds1–17as other methodological information are reported in theSupplementary Methods. Figure 3: Structure of potential pre-substrates 1–3 and S1-binding fragments 4–17. The details of the synthesis of compounds 1–17 as other methodological information are reported in the Supplementary Methods . Full size image Screening with different nucleophiles All fragments were investigated separately at identical concentrations on 96-well microtitre plates with and without one of the proteases for activation of the three pre-substrates. No increase of fluorescence was observed for any of the fragments together without protease in the reaction buffer. In situ formation of substrates by dynamic ligation of a fragment and a pre-substrate was detected via release of the fluorescent reporter molecule, AMC by amide bond cleavage. AMC-release was followed by excitation at 380 nm and fluorescence detection at 460 nm. The fluorescence intensity at 460 nm was recorded in each well for a time period of 15 min and the slope was determined for a comparison of all fragment–pre-substrate combinations. For each of the three pre-substrates, several activating fragments were identified, whereas none of the pre-substrates was activated by one of the negative control fragments 14–16 . Glyoxalyl-AMC 1 was activated by 9 out of 14 fragments to a substrate of trypsin, and by 7 out of 14 fragments to a substrate of FXa. 9 (ethanolamine), 7 (butane-1,4-diamine), 11 (4-(aminomethyl)benzamidine) and 4 (2-hydroxyethylguanidine) were found to be most active for 1 and trypsin ( Table 1 , entry 6, 4, 7 and 1), whereas ethanolamine 9 , 2-hydroxyethylguanidine 4 and butane-1,4-diamine 7 were established as the most active molecules for 1 and FXa ( Table 1 , entry 6, 1 and 4). Malonalyl-AMC 2 was turned into a trypsin substrate by 11 out of 14 non-control fragments, and into a FXa substrate by 10 fragments. In the presence of trypsin, 2 was best activated by fragments 6 and 9 ( Table 1 , entry 3 and 6); in the presence of FXa by fragments 4 , 9 and 11 ( Table 1 , entry 1, 6 and 7). In general, as summarized in Table 1 , both the activating effect of different nucleophiles varied between the pre-substrates and between the two proteases ( Supplementary Figs 5 and 7 ). Glyoxalyl-AMC was most efficiently activated towards trypsin by the hydroxy-derivatives of the Lys and arginine mimetics, followed by the diamines (forming Lys isosters) and then the amino-substituted guanidines (forming Arg isosters). FXa was more selective in the acceptance of fragments (and ligation products), and had distinct preferences with respect to the strength of activation. Table 1 Quantitative determination of pre-substrate activation. Full size table Next, a quantitative description of the observed activation of pre-substrates by nucleophilic fragments and of the templating effect exerted by the enzymes was to be established. For the purpose, a modified Michaelis–Menten model for enzymatic reactions was adapted to the special case of pre-substrate activation. In this model, the protease P was expected to bind a nucleophilic fragment F in its S1 pocket, which reacted in a dynamic and covalent ligation reaction to form the three-component protease–fragment–pre-substrate (P–F–PS) complex. Taking into account the S1 affinity of the employed nucleophiles and the non-detectable binding of the pre-substrates to the protein alone, one can assume that the binding of the nucleophilic fragment is the initial step of the complex formation. The P–F–PS complex is then converted by the enzyme yielding free AMC as the detectable product. Experimentally, the rate of the enzymatic reaction, V , corresponding to the cleavage of the ligation product can be determined. When V was measured at a fixed pre-substrate concentration (3 mM), the saturation of the reaction rate to V max could be determined for increasing fragment concentrations. The fragment concentration at the half maximal rate ( V max /2) was considered as the apparent K M value ( K M *) of the ligation product and indicates the stability of the enzyme–ligation product complex, the P–F–PS complex ( Fig. 4 ). 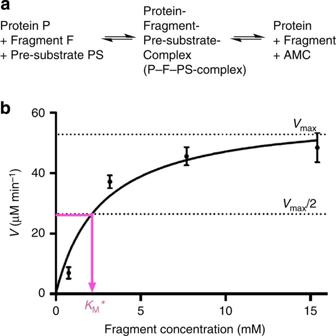Figure 4: Model for the activation of pre-substrates by nucleophilic protein-binding fragments. One protease molecule, a fragment and a pre-substrate form a three-component P–F–PS complex, which releases the coumarin dye AMC as a result of the enzymatic activity of the protease (a). The apparentKMvalue, reflecting the stability of the P–F–PS complex, can be derived from the half maximal rate of the enzymatic reactionVmax/2 as exemplified here for the combination of protease FXa, fragment7and pre-substrate1(b). Figure 4: Model for the activation of pre-substrates by nucleophilic protein-binding fragments. One protease molecule, a fragment and a pre-substrate form a three-component P–F–PS complex, which releases the coumarin dye AMC as a result of the enzymatic activity of the protease ( a ). The apparent K M value, reflecting the stability of the P–F–PS complex, can be derived from the half maximal rate of the enzymatic reaction V max /2 as exemplified here for the combination of protease FXa, fragment 7 and pre-substrate 1 ( b ). Full size image It should be noted that the thermodynamic stabilization of the P–F–PS complex expressed as K M * value is a direct measure for the templating effect exerted by the enzyme, which corresponds to the free energy of complex formation and describes the shift in the equilibrium from the free fragments to the ligated fragments. Determinations of both K M and V max values were conducted for the seven most active fragments, two pre-substrates and two enzymes ( Table 1 ). The apparent K M values of the three-component P–F–PS complexes varied between 130 μM (for the combination of PS 2 , F 9 and FXa as protease) and ca. 6 mM (for the combination of PS 1 , F 6 and trypsin). The V max values were between 12.9 μM min −1 (PS 1 , F 4 and FXa) and 242.3 μM min −1 for the combination of PS 2 , F 7 and FXa. No stringent correlation between the K M and V max values was observed for both enzymes and pre-substrates, however, in most of the cases, the V max was higher with PS 2 ; in 11 out of 14 cases it was more than twofold. The kinetic analysis of pre-substrate activation revealed that the reaction process was catalytic in a double sense. Not only the proteases but also the nucleophilic fragments themselves acted as catalysts in the conversion of the pre-substrate without being consumed or modified in the process. While the catalytic action of proteases as enzymes was expected, the organo-catalytic effect [36] , [37] of the protein-binding nucleophile was remarkable, as it constitutes to our best knowledge the first example of a catalytic activity of a small molecule in a protein-templated reaction. Michael addition ligation The third pre-substrate, N -acrylamido-AMC 3 , was selected as a model for irreversible pre-substrate activation. Activation of 3 was investigated in the presence of thiol nucleophiles, which were expected to yield Michael addition products being stable under assay conditions [38] , [39] . Thus, pre-substrate 3 was incubated with one of three thiol nucleophiles, 2-mercaptoethyl-guanidine 6 , cysteamine 10 and 4-amino benzenethiol in the assay buffer for 30 min at room temperature (20 °C). Subsequently, trypsin was added and time-dependent fluorescence was recorded at 480 nm ( Fig. 5 ). The thiol fragments 6 and 10 were active and led to the release of AMC, while no activation was observed with the negative control fragment, 4-aminobenzenethiol. For an independent confirmation of the observed pre-substrate activation, the Michael addition product 18 , formed by reaction of cysteamine 10 and presubstrate 3 was synthesized at 35 °C ( Supplementary Fig. 4 ), isolated and tested in the presence of trypsin. leading to a comparable release of AMC ( Fig. 5 , method B). Thus, it has been demonstrated that the activation of pre-substrates can be effected not only by reversible but also by irreversible ligation reactions. 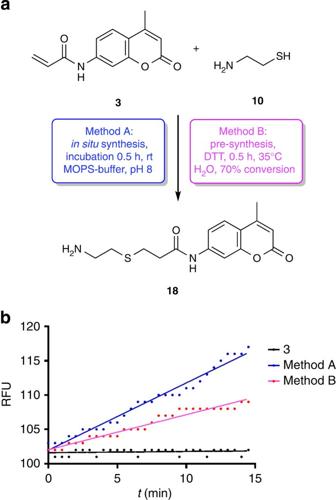Figure 5: Activation of pre-substrate 3. (a) Reaction scheme. (b) Recorded fluorescence of released AMC over time. Influence of ligation product (in situformed from3and10, method A, blue) in comparison with isolated substrate18on the enzyme activity (method B, magenta). The experiments were repeated twice by two different operators with duplicates measured within each replication. Each data point represents the average of double determination. DTT, 1,4-dithio-D-threitol; rt, room temperature. Figure 5: Activation of pre-substrate 3. ( a ) Reaction scheme. ( b ) Recorded fluorescence of released AMC over time. Influence of ligation product ( in situ formed from 3 and 10 , method A, blue) in comparison with isolated substrate 18 on the enzyme activity (method B, magenta). The experiments were repeated twice by two different operators with duplicates measured within each replication. Each data point represents the average of double determination. DTT, 1,4-dithio-D-threitol; rt, room temperature. Full size image Three-fragment assembly Finally, it was investigated, if the pre-substrate concept could be extended further from two-fragment assemblies as demonstrated above to the protein template-assisted formation of bioactive assemblies consisting of three-components. This investigation was based on the following consideration. Pre-substrate 2 was found to be activated efficiently by butane-1,4-diamine 7 . If one assumes that this activation proceeds via formation of the amino-butyl-imine 19 as the substrate and reversibly formed two-fragment assembly, one can hypothesize that a third fragment might be able to add to the imine 19, yielding an assembly of three fragments with potentially enhanced substrate activation ( Fig. 6 ). To test this hypothesis, fragment 7 was incubated with one of the two proteases (trypsin or FXa), pre-substrate 2 and either 6 or 10 as third fragments. As described above, fragment 6 , 7 and 10 activated the pre-substrate 2 when added as secondary fragment. Addition of the third fragment generated for both enzymes and for both thiol fragments stronger AMC fluorescence. For trypsin, the strongest activation of pre-substrate 2 was observed with fragments 7 and 10 by 56% or 50 relative fluorescence units (RFUs) after 15 min ( Fig. 6a ); for FXa, the combination of 2 with 7 and 6 resulted in the strongest activation by almost 100% or 80 RFU after the same time ( Fig. 6b ). In both cases, the activation by three fragments was compared with activation of a doubled concentration of fragment 7 (15 mM instead of 7.5), which yielded no or low increase in fluorescence, indicating that there was indeed an enhancing effect of the third fragment added. 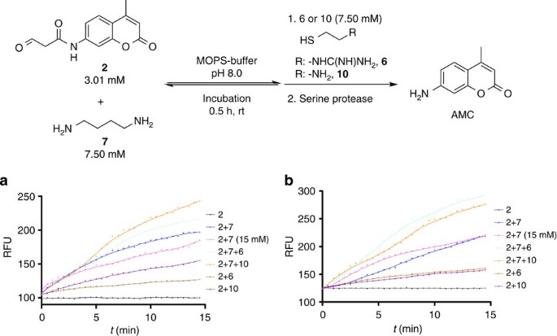Figure 6: Three-fragment assembly. Influence of nucleophilic fragments7,6and10and pre-substrate2on the enzyme activity; (a) trypsin, (b) factor Xa. The experiments were replicated twice by two different operators. Each data point represents the average of double determination. Figure 6: Three-fragment assembly. Influence of nucleophilic fragments 7 , 6 and 10 and pre-substrate 2 on the enzyme activity; ( a ) trypsin, ( b ) factor Xa. The experiments were replicated twice by two different operators. Each data point represents the average of double determination. Full size image It has been demonstrated that protein-binding small molecule fragments can induce chemical reactions on the protein surface in a catalytic process. Nucleophilic, low molecular weight fragments binding to the S1 pocket of serine proteases were able to activate electrophilic pre-substrates in a protein-templated reaction. Activation of pre-substrates occurred via a dynamic covalent ligation reaction on the protein surface and both the free nucleophile and the presence of the enzyme were essential for this process. The reversible ligation reaction of the protein-bound amino-, hydroxy-, or mercapto-nucleophile with the electrophile positioned the pre-substrate into the active site of the enzyme and thereby induced the enzymatic hydrolysis of the protein–fragment–pre-substrate assembly. The activation process was studied quantitatively with three pre-substrates containing N -acylated AMC as a fluorogenic dye, which upon hydrolysis released the fluorophore 7-amino-methyl coumarin. The cleavage reaction was monitored by fluorescence spectrometry. The mechanism of pre-substrate activation was confirmed by the results of several control experiments. Only S1-binding fragments containing a free nucleophile available for dynamic covalent ligation were able to activate pre-substrates. No cleavage of the pre-substrate was observed without presence of a protease. Second, HPLC analysis of the assay solution revealed that the increase in fluorescence indeed correlated with the hydrolytic cleavage of pre-substrates and the release of 7-amino-methyl coumarin. The rate of the pre-substrate cleavage ( V ) was measured as a function of the fragment concentration for all combinations of one of eight active fragments with one of two pre-substrates and proteases. In all cases, the substrate cleavage rate V increased with growing fragment concentrations and could be saturated when approaching the maximal conversion rate ( V max ). The stability of the protease–fragment–pre-substrate (P–F–PS) complex, K M * , was determined for each of the tested P–F–PS combinations as the fragment concentration at the half maximal velocity ( V max /2). The stability of the P–F–PS complex is a direct measure for the free enthalpy of complex formation and thus the K M * values indicate quantitatively the shift in the ligation equilibrium exerted by the enzyme’s templating effect. Both the V max and the K M * values were specific for each of the tested P–F–PS combinations, suggesting both a specific recognition effect exerted by the protease and a specific catalytic activation effect of the bis-nucleophile. No correlation between the stability of the P–F–PS complex and the maximal cleavage rate was observed, however, the cleavage rates were consistently higher for pre-substrate 2 compared with pre-substrate 1 , suggesting that the latter compound ensures—at least for the activating fragments tested here—a better positioning of the cleaved amide bond in the active site of the enzyme. The pre-substrate concept was further extended from reversible towards irreversible, covalent fragment ligations as demonstrated with the Michael addition of thiol nucleophiles to the acrylamide containing pre-substrate 3 . Finally, pre-substrate activation was conducted not only by dimeric ligations (with two fragments) but also using hetero-trimeric fragment assemblies, if one amine and one thiol nucleophile were employed. The reported activation of pre-substrates constitutes a novel approach to identify small molecule fragments binding specifically to defined protein-binding pockets. The described assays—demonstrated here for the S1-pockets of two proteases, trypsin and FXa—enable the quantitative detection of protein-templated ligation reactions. The templating effects responsible for shifting the ligation equilibrium can be determined quantitatively. One would further expect that the activation of pre-substrates can be applied to other proteases as well and can be extended towards other secondary binding sites and towards other classes of hydrolytic enzymes, whenever a protein-bound primary fragment is capable to react with a secondary fragment and thereby direct cleavable bond at the active site of the protein. The assays can be extended to the screening of larger libraries of nucleophilic fragments and the sensitized detection of fragments binding to defined pockets of enzymes might serve as a starting point for the development of site-directed inhibitors of these enzymes as well. Libraries of nucleophilic fragments are smaller and less diverse than unbiased fragment libraries. On the other hand, presence of a nucleophilic functionality in all hits of a pre-substrate screen will facilitate the subsequent extension of hit fragments, possibly in an iterative ligation screening step. Beyond its practical implications, pre-substrate activation by protein-binding nucleophiles constitutes an example for a coupling of dynamic covalent ligation reaction with an enzymatic reaction. The protein-binding nucleophilic fragments act as organo-catalysts for the hydrolysis of the pre-substrate by the enzyme. Such organo-catalytic reactions of protein-binding fragments in fact enlarge the substrate pool of enzymes by pre-substrates and thereby extend the realm of exploitable enzymatic reactions. General methods The details of the synthesis of compounds 1 – 18 ( Supplementary Figs 1–4 ) as other methodological information are reported in the Supplementary Methods . The activity of the serine proteases was determined by measuring the release of AMC from the fluorogenic substrate synthesized in situ on 96-well microtitre plates using a Tecan Safire 2 wellplate reader. The excitation wavelength was set to 380 nm and emission was recorded at 460 nm. For the analysis of the data, GraphPad Prism 5 was used. Purity characterization of trypsin and FXa and also the investigation of side reactions between pre-substrate and proteins were analyzed using MALDI-MS. MALDI-ToF/ToF MS was performed on Ultraflex III, Bruker Daltonics 2007 equipped with a smartbeam laser (Nd:YAG). SDHB (mixture of 2,5-dihydroxybenzoic acid and 2-hydroxy-5-methoxybenzoic acid) or CA (alpha-cyano-4-hydroxycinnamic acid) from Bruker Daltonics were used as matrix materials. Buffers and reagents were purchased from Roth and Sigma-Aldrich. Water was purified by ultrafiltration (Millipore Simplicity 185). Human FXa was obtained as lyophilized powder by Enzyme Research Laboratories Ltd (Catalogue: HFXa 1011, activity: 228 IU mg −1 ) and dissolved in BisTris-buffer (bis(2-hydroxyethyl)amino-tris(hydroxymethyl)methane, pH 6). Bovine trypsin was acquired by Sigma-Aldrich as lyophilized powder (T1426 Sigma, TPCK treated, essentially salt free, >100,000 BAEE U mg −1 protein) and taken up in 1 mM HCl. MOPS-NaOH buffer pH 8 was prepared in ultra pure water. 3-( N -morpholino)-propanesulfonic acid (MOPS, 50 mM) and NaCl (154 mM) were dissolved in water; pH was adjusted with NaOH (stored at 4 °C). DLS procedures First procedure . Pre-substrate activation by nucleophilic protein-binding fragments. First screening procedure was performed using the pre-substrate 1 or 2 (3 μl of 233 mM stock solution in DMSO resulting in 3.07 mM assay concentration) and one of the various nucleophilic fragments 4 – 17 (3 μl of 0, 60, 240, 580 or 1,160 mM stock solution in DMSO resulting in 0, 0.77, 3.2, 7.7 or 15.4 mM assay concentration) in a total volume of 206 μl MOPS-NaOH buffer (pH 8, 50 mM) per well. Fluorescence was monitored starting immediately after the addition of 20 μl of the serine protease solution (3.5 nM trypsin or 3.5 nM FXa; 1/1,000 dilution in bovine serum albumin (BSA) 0.1% (wt/vol), NaCl 154 mM). The initial rates were determined and plotted against the fragment concentration ( Supplementary Figs 5 and 7 ). Second procedure . Three-fragment assembly screening. The three-fragment assembly screening was investigated using pre-substrate 2 (3 μl of 233 mM DMSO stock solution equates to 3.07 mM assay concentration) and fragment 7 (3 μl of 580 or 1,160 mM DMSO stock solution equates to 7.7 mM or 15.4 mM assay concentration) in a total volume of 206 μl MOPS-NaOH buffer (pH 8, 50 mM). After incubation (30 min, room temperature) the second nucleophilic fragment 6 or 10 (3 μl of 580 mM DMSO stock solution equates to 7.7 mM assay concentration; Fig. 2 , Part b) and 20 μl of the serine protease solution (3.5 nM trypsin or 3.5 nM FXa; dilution in BSA 0.1% (wt/vol), NaCl 154 mM) was added. The fluorescence intensities were plotted over time ( Fig. 6 ). Third procedure . Michael addition screening. Third screening procedure was performed using pre-substrate 3 (3 μl of 233 mM DMSO stock solution equates to 3.07 mM assay concentration) and cysteamine 10 (3 μl of 580 mM DMSO stock solution equates to 7.7 mM assay concentration) in a total volume of 206 μl MOPS-NaOH buffer (pH 8, 50 mM). After incubation (30 min, 35 °C) 20 μl serine protease (3.5 nM trypsin or 3.5 nM FXa; dilution in BSA 0.1% (wt/vol), NaCl 154 mM) was added. Relative fluorescence was recorded and plotted against the time ( Fig. 5 ). For comparison the addition product 18 was pre-synthesized. Twenty microlitres of serine protease (3.5 nM trypsin or 3.5 nM FXa; dilution in BSA 0.1% (wt/vol), NaCl 154 mM) was added to the isolated compound 18 (5 μl of 140 mM DMSO stock solution equates to 3.01 mM assay concentration) in a total volume of 205 μl MOPS-NaOH buffer (pH 8, 50 mM). The measurement was started without secondary incubation. Determination of RFUs For the determination of RFUs, the fluorescence of AMC was measured at different concentrations. RFUs (RFUs; λ 460 nm) were found to correlate linearly with the AMC concentration at concentration between 0 and 8 mM. The calculation factor was determined as being 47.465 RFU per μM AMC and the initial rates in μM min −1 were plotted against the fragment concentrations ( Supplementary Fig. 6 ). HPLC investigations Twenty microlitres of trypsin (3.5 nM; dilution in BSA 0.1% (wt/vol), NaCl 154 mM) was added to pre-substrate 1 (20 μl of 4 mM stock solution equates to 0.307 mM assay concentration) and fragment 4 (20 μl of 12 mM stock solution equates to 0.92 mM assay concentration) in total volume of 240 μl distilled water and mixed over 0, 5 and 25 min. Next, 260 μl acetonitrile was added to the probes, mixed and analyzed by HPLC. The turnover frequency (TOF) refers to the trypsin and was calculated on the basis of the amount of the product formed as well as the amount of trypsin used per minute. The reaction was detected at 340 and 430 nm ( Supplementary Fig. 8 ). MALDI-TOF/TOF MS investigations Purity characterizations . Trypsin (10.2 μM; dilution in water) and FXa (42.6 μM; dilution in water) were analyzed separately with SDHB (mixture of 2,5-dihydroxybenzoic acid and 2-hydroxy-5-methoxybenzoic acid) or cinnamic acid (CA) matrix material ( Supplementary Figs 9 and 10 ). Investigation of side reactions between trypsin and pre-substrate 1 . Twenty microlitres of trypsin (10.2 μM, dilution in water) was incubated with 2 μl pre-substrate 1 (100 μM, dilution in water). The reaction mixture was analyzed using CA matrix material. Investigation of side reactions between trypsin, pre-substrate 1 and fragment 4 . Twenty microlitres of trypsin (10.2 μM, dilution in water) was incubated with 2 μl pre-substrate 1 (100 μM, dilution in water) and 2 μl fragment 4 (100 μM, dilution in water). The reaction mixture was analyzed using CA matrix material; ( Supplementary Fig.11 ). How to cite this article: Burda, E. and Rademann, J. Catalytic activation of pre-substrates via dynamic fragment assembly on protein templates. Nat. Commun. 5:5170 doi: 10.1038/ncomms6170 (2014).